A high-energy-density sugar biobattery based on a synthetic enzymatic pathway High-energy-density, green, safe batteries are highly desirable for meeting the rapidly growing needs of portable electronics. The incomplete oxidation of sugars mediated by one or a few enzymes in enzymatic fuel cells suffers from low energy densities and slow reaction rates. Here we show that nearly 24 electrons per glucose unit of maltodextrin can be produced through a synthetic catabolic pathway that comprises 13 enzymes in an air-breathing enzymatic fuel cell. This enzymatic fuel cell is based on non-immobilized enzymes that exhibit a maximum power output of 0.8 mW cm −2 and a maximum current density of 6 mA cm −2 , which are far higher than the values for systems based on immobilized enzymes. Enzymatic fuel cells containing a 15% (wt/v) maltodextrin solution have an energy-storage density of 596 Ah kg −1 , which is one order of magnitude higher than that of lithium-ion batteries. Sugar-powered biobatteries could serve as next-generation green power sources, particularly for portable electronics. The rapidly growing demand for powering portable electronic devices is driving the development of better batteries with features such as enhanced energy-storage densities, high levels of safety, fast rechargeability, biodegradability and small environmental footprints [1] . The rechargeable lithium-ion battery is often the system of choice because it offers a high energy density, has a flexible and light-weight design and has a longer lifespan than comparable battery technologies [1] , [2] . The energy-storage density of a typical lithium-ion battery is ~0.54 MJ kg −1 (that is, 150 Wh kg −1 ). The widespread use of metal-catalysed batteries also raises many concerns, primarily related to safety, toxic metal pollution and the availability of costly, limited, irreplaceable or rare metal resources. Enzymatic fuel cells (EFCs) are emerging electrobiochemical devices that directly convert chemical energy from a variety of fuels into electricity using low-cost biocatalyst enzymes [3] , [4] , [5] , [6] . Inspired by living cells that can utilize complex organic compounds, for example, starch and glycogen) as stored energy sources, sugar-powered EFCs represent the next generation of biodegradable, highly safe biobatteries. Compared with microbial fuel cells, EFCs usually generate much higher power density in terms of mW cm −2 . This feature highlights their great potential for powering a variety of portable electronic devices in the near future [5] , [7] , [8] . In principle, fuels used in EFCs can have high energy-storage densities if they are completely oxidized. For example, the combustion energy of glucose is 15.5 MJ kg −1 . Glucose can release up to 3,574 Ah kg −1 , which is 85-fold greater than the energy released by lithium-ion batteries (42 Ah kg −1 ). Most EFCs run on complex organic compounds (for example, glucose, methanol, glycerol and so on). Therefore, high energy-storage density potentials can only be achieved if these fuels are completely oxidized to CO 2 , as occurs in living cells through complicated catabolic pathways. However, natural catabolic pathways may not be feasible for practical use in EFCs, because nearly all of these pathways require costly and labile reagents, such as ATP, coenzyme A and complex cellular membranes. The incomplete oxidation of organic fuels mediated by one or a few enzymes in EFCs results in low energy densities, waste of fuel and inhibition of enzymes by the metabolic products. In vitro synthetic enzymatic pathways have been constructed on the anode compartments in EFCs for deep or complete oxidation of methanol [9] , [10] , ethanol [11] , glycerol [12] and glucose [13] . However, previous studies did not provide quantitative evidence (for example, Faraday efficiency) for the complete oxidation of organic fuels in microbial fuel cells [14] , [15] . Sugars are appealing fuels for EFCs because they are abundant, renewable, inexpensive in terms of $ GJ −1 , non-toxic, safe for storage and distribution, and carbon neutral over the entire life cycle [16] . Starch is the most widely used energy-storage compound in nature. The catabolism of starch allows for a slow and nearly constant release of chemical energy in living cells that is different from its monomer glucose [17] . Maltodextrin, a partially hydrolysed starch fragment, is a superior fuel to glucose in EFCs, because maltodextrin has 11% higher energy density than glucose. Maltodextrin is also less costly because glucose is the main product of its enzymatic hydrolysis, and low-cost linear maltodextrin can be made from cellulose [17] . An equivalent weight of maltodextrin has a much lower osmotic pressure than glucose. Moreover, it can provide slowly metabolized glucose-1-phosphate for more stable electricity generation in closed EFCs [6] . Maltodextrin has been used as a fuel for EFCs, but only two electrons could be generated per glucose unit [6] . In this study, a synthetic ATP- and CoA-free catabolic pathway that comprises 13 enzymes in an air-breathing EFC is constructed to completely oxidize the glucose units of maltodextrin, yielding nearly 24 electrons per glucose. We find that the EFC based on non-immobilized enzymes exhibits a maximum power output far higher than those based on the immobilized enzymes. These sugar-powered biobatteries feature high energy-storage densities and high safety. Thus, these batteries represent next-generation micropower sources that could be especially useful for portable electronics. Comparison of non-immobilized and immobilized enzymes Enzyme immobilization on the surface of conductive electrodes is widely used in nearly all EFCs. Enzymes are immobilized using a variety of methods, including gel entrapment, physical adsorption, chemical covalent linking and immobilization with nanoparticles and nanotubes [3] , [18] , [19] . These methods originated from biosensors that focus on achieving reproducible signals by immobilizing commercially available mesophilic enzymes to enhance their stability without concern for slow reaction rates [3] , [20] . However, enzymes immobilized on the surface of solid electrodes generally exhibit much lower activities (for example, 1%) due to enzyme deactivation and poor fuel transfer from the bulk solutions to the immobilized enzymes [8] , [21] , [22] . To achieve constant high-power EFCs, we considered an alternative strategy for mediating electron transfer in the EFCs without immobilizing the enzymes. Our strategy retains the enzymatic activity and facilitates mass transfer by immobilizing the electron mediator (that is, vitamin K 3 (VK 3 )) on the surface of the electrode ( Fig. 1a(3) ). The stability of enzymes can be addressed by the use of thermoenzymes. In this study, the thermoenzymes were produced in E. coli and purified by three methods: heat precipitation, His-tag/nickel charged resin and adsorption of cellulose-binding-module-tagged proteins on a cellulosic adsorbent ( Supplementary Fig. S1 and Supplementary Table S1 ). Two typical enzyme immobilization approaches for EFCs were used as controls: polymer matrix entrapment in a quaternary tetrabutylammonium bromide (TBAB)-modified Nafion [11] ( Fig. 1a(1) ) and covalent binding on carbon nanotubes (CNTs) [23] ( Fig. 1a(2) ). To compare the EFCs equipped with non-immobilized enzymes with the two EFCs equipped with immobilized enzymes, equivalent amounts of glucose-6-phosphate (g6p) dehydrogenase (G6PDH) and diaphorase (DI) were used to test the polarization and the power outputs of the EFCs for g6p fuel ( Fig. 1b,c ). The mass transport region for the non-immobilized EFCs occurred at higher current densities compared with the covalent binding-based EFCs ( Fig. 1b ), suggesting the influence of enhanced mass transport for the non-immobilized enzymes. The EFC based on non-immobilized G6PDH exhibited the highest power density of 0.13 mW cm −2 , three times higher than that of the covalent binding method. The EFC based on the TBAB-modified Nafion polymer entrapment method had the lowest maximum power density of 0.0013, mW cm −2 , which was only 4% of the density for the covalent binding method. The G6PDH immobilized by Nafion polymer entrapment and the covalent binding retained 0.2 and 6% of its non-immobilized activity, respectively. The DI immobilized by Nafion polymer entrapment and the covalent binding retained 0.4% and 7.5% of its non-immobilized activity, respectively ( Supplementary Table S2 ). These data for enzyme activity clearly suggest that a dramatic activity loss occurs due to enzyme immobilization [21] , [22] . The power density data validate the feasibility of using non-immobilized enzyme(s) to achieve high-power output in EFCs. 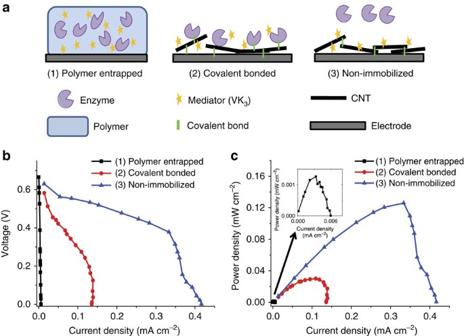Figure 1: Comparison of electrodes based on immobilized and non-immobilized enzymes. (a) Schematic of (1) the TBAB-modified Nafion polymer-entrapped immobilization, (2) the covalent bonded CNT immobilization and (3) the non-immobilized enzymes. Profiles of voltage versus current density (b) and of power density versus current density (c) using (1) the TBAB-modified Nafion polymer-entrapped immobilization (inserted figure), (2) the covalent bonded immobilization and (3) the non-immobilized enzymes. The experimental conditions were 1 U of G6PDH, 40 U of DI, 10 mM g6p in the 100 mM HEPES (pH 7.5) buffer containing 2 mM NAD+, 10 mM MgCl2and 0.5 mM MnCl2at room temperature. Figure 1: Comparison of electrodes based on immobilized and non-immobilized enzymes. ( a ) Schematic of (1) the TBAB-modified Nafion polymer-entrapped immobilization, (2) the covalent bonded CNT immobilization and (3) the non-immobilized enzymes. Profiles of voltage versus current density ( b ) and of power density versus current density ( c ) using (1) the TBAB-modified Nafion polymer-entrapped immobilization (inserted figure), (2) the covalent bonded immobilization and (3) the non-immobilized enzymes. The experimental conditions were 1 U of G6PDH, 40 U of DI, 10 mM g6p in the 100 mM HEPES (pH 7.5) buffer containing 2 mM NAD + , 10 mM MgCl 2 and 0.5 mM MnCl 2 at room temperature. Full size image Complete oxidation of maltodextrin To release the maximum electron potential from each glucose unit (that is, 24 per glucose), we designed a non-natural enzymatic pathway containing 13 enzymes ( Fig. 2a ). This synthetic pathway consists of four functional modules: g6p generation from maltodextrin mediated by α-glucan phosphorylase (α-GP) and phosphoglucomutase (PGM) (equation 1); two reduced NADH generated from g6p mediated by two NAD-dependent G6PDH and 6-phosphogluconate dehydrogenase (6PGDH) (equation 2); NADH electro-oxidation through non-immobilized DI to immobilized VK 3 that generates 2 electrons per NADH (equation 3); and 5/6 moles of g6p regeneration from 1 mole of ribulose-5-phosphate via a hybrid pathway that comprises enzymes in the pentose phosphate, glycolysis and gluconeogenesis pathways (equation 4). The overall anode reaction for the combination of equations 1, 2, 3, 4 approximately results in equation 5. Clearly, each glucose unit from maltodextrin can generate 24 electrons on the anode via this de novo pathway (equation 5). 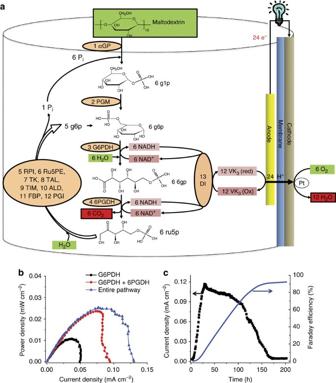Figure 2: Complete oxidation of maltodextrin based on a synthetic enzymatic pathway. (a) Schematic of the complete oxidation of maltodextrin via the synthetic catabolic pathway. The enzymes are as follows—1: αGP, α-glucan phosphorylase; 2: PGM, phosphoglucomutase; 3: G6PDH, glucose-6-phosphate dehydrogenase; 4: 6PGDH, 6-phosphogluconate dehydrogenase; 5: RPI, ribose-5-phosphate isomerase; 6: Ru5PE, ribulose-5-phosphate 3-epimerase; 7: TK, transketolase; 8: TAL, transaldolase; 9: TIM, triosephosphate isomerase; 10: ALD, aldolase; 11: FBP, fructose-1,6-bisphosphatase; 12: PGI, phosphoglucose isomerase; and 13: DI, diaphorase. The key metabolites are glucose-1-phosphate (g1p), glucose-6-phosphate (g6p), 6-phosphogluconate (6 pg) and ribulose-5-phosphate (ru5P). Pi, inorganic phosphate; VK3, vitamin K3. (b) Profiles of power density versus current density for the sugar biobattery using only G6PDH, G6PDH and 6PGDH, or the entire pathway. The experimental conditions were 100 mM HEPES, pH 7.5, buffer containing 0.1 mM maltodextrin, 4 mM NAD+, 100 mM HEPES, pH 7.5, 4 mM sodium phosphate, 10 mM MgCl2, 0.5 mM MnCl2, 5 mM DTT and 0.5 mM thiamine pyrophosphate at room temperature. The enzyme loading conditions are shown inSupplementary Table S1. (c) Profiles for current generation and cumulative Faraday efficiency. The experimental conditions were 100 mM HEPES, pH 7.5, buffer containing 0.1 mM of maltodextrin, 10 mM MgCl2, 0.5 mM MnCl2, 4 mM NAD+, 4 mM sodium phosphate, 5 mM DTT, 0.5 mM thiamine pyrophosphate, 50 mg l−1kanamycin, 40 mg l−1tetracycline, 40 mg l−1cycloheximide, 0.5 g l−1sodium azide, 1 g l−1BSA and 0.1% Triton X-100. Figure 2: Complete oxidation of maltodextrin based on a synthetic enzymatic pathway. ( a ) Schematic of the complete oxidation of maltodextrin via the synthetic catabolic pathway. The enzymes are as follows—1: αGP, α-glucan phosphorylase; 2: PGM, phosphoglucomutase; 3: G6PDH, glucose-6-phosphate dehydrogenase; 4: 6PGDH, 6-phosphogluconate dehydrogenase; 5: RPI, ribose-5-phosphate isomerase; 6: Ru5PE, ribulose-5-phosphate 3-epimerase; 7: TK, transketolase; 8: TAL, transaldolase; 9: TIM, triosephosphate isomerase; 10: ALD, aldolase; 11: FBP, fructose-1,6-bisphosphatase; 12: PGI, phosphoglucose isomerase; and 13: DI, diaphorase. The key metabolites are glucose-1-phosphate (g1p), glucose-6-phosphate (g6p), 6-phosphogluconate (6 pg) and ribulose-5-phosphate (ru5P). P i , inorganic phosphate; VK 3 , vitamin K 3 . ( b ) Profiles of power density versus current density for the sugar biobattery using only G6PDH, G6PDH and 6PGDH, or the entire pathway. The experimental conditions were 100 mM HEPES, pH 7.5, buffer containing 0.1 mM maltodextrin, 4 mM NAD + , 100 mM HEPES, pH 7.5, 4 mM sodium phosphate, 10 mM MgCl 2 , 0.5 mM MnCl 2 , 5 mM DTT and 0.5 mM thiamine pyrophosphate at room temperature. The enzyme loading conditions are shown in Supplementary Table S1 . ( c ) Profiles for current generation and cumulative Faraday efficiency. The experimental conditions were 100 mM HEPES, pH 7.5, buffer containing 0.1 mM of maltodextrin, 10 mM MgCl 2 , 0.5 mM MnCl 2 , 4 mM NAD + , 4 mM sodium phosphate, 5 mM DTT, 0.5 mM thiamine pyrophosphate, 50 mg l −1 kanamycin, 40 mg l −1 tetracycline, 40 mg l −1 cycloheximide, 0.5 g l −1 sodium azide, 1 g l −1 BSA and 0.1% Triton X-100. Full size image The pathway utilizes two NAD-dependent G6PDH and 6PGDH to generate NADH differently from natural NADP-dependent enzymes in the pentose phosphate pathway used for anabolism. The above pathway does not require either ATP or CoA, which are very costly and unstable in EFCs [11] , [24] . Moreover, phosphate ions can be recycled to maintain constant pH and ion concentrations. This cyclic pathway design is different from the linear pathways typically used in EFCs [9] , [12] , [13] . The power densities from maltodextrin fuel (that is, 2 mM glucose units) were compared for three EFCs that used one dehydrogenase (that is, G6PDH), two dehydrogenases (that is, G6PDH and 6PGDH) or the entire pathway ( Fig. 2b ). The open circuit potentials were similar for the three EFCs (~0.7 V). When only G6PDH was used, the EFC exhibited a maximum power density of 0.011 mW cm −2 . When a second dehydrogenase (6PGDH) was added, the maximum power density increased by a factor of 2, to 0.024 mW cm −2 . When eight additional enzymes were added to reconstitute the entire pathway ( Fig. 2a ), the maximum power density increased slightly to 0.026 mW cm −2 . The corresponding maximum current density was 35% higher than the current density of the system based on two dehydrogenases ( Fig. 2b ). To quantitatively validate the complete oxidation of the glucose units of maltodextrin, we measured the Faraday efficiency from NADH to electrons through the DI and VK 3 in the air-breathing EFC ( Supplementary Fig. S2 ). Under oxygen-free conditions for the anode compartment, the Faraday efficiency of the EFC was 97.6±3.0% ( Supplementary Fig. S3 ), suggesting that the electro-enzymatic oxidation of NADH is highly efficient [9] . Moreover, the removal of oxygen from the anode compartment was essential for obtaining a high Faraday efficiency and preventing the non-selective oxidation of NADH. In a 15-mL EFC containing 13 enzymes and a low concentration of maltodextrin at room temperature ( Fig. 2c ), the current density increased to a peak value of 0.12 mA cm −2 at 24 h and then decreased slowly due to substrate consumption. After >150 h, the current output decreased to nearly zero. The cumulative electric charge generated was 48.9 C relative to the theoretical electric charge generated based on the consumption of the glucose units (that is, 53.0 C, 1 mole of glucose unit can generate 24 × 96,485 C in principle). This result suggests a cumulative Faraday efficiency of 92.3% with 1 mole of glucose generating 22.2 moles of electrons. It was noted that the negative control (that is, the same EFC without the substrate) did not generate significant current outputs ( Supplementary Fig. S4 ). The Faraday efficiency was higher than that of the microbial fuel cell based on glucose (83%) [14] , because cell-free biosystems do not waste organic fuels on cell growth and byproduct formation, as demonstrated previously [25] , [26] . Our system provides the first quantitative evidence for nearly 24 electrons produced per glucose unit in an EFC. Moreover, our data suggest that we can convert all of the chemical energy from the sugar into electrical energy and increase the energy density of the EFC by one order of magnitude. High-energy-density high-power EFCs Power density is another important consideration in EFCs. To increase the power density, we optimized a number of factors, including the EFC configuration, the enzyme loading and the experimental conditions under which the non-immobilized G6PDH acts on g6p. The optimal CNT loading was 3 mg cm −2 of carbon paper ( Supplementary Fig. S5a ). The six electrodes stacked together as a three-dimensional anode increased the maximum power density by 50% and the maximum current density by fourfold ( Supplementary Fig. S5a,b ). Increasing the enzyme loading from 1 to 10 U per cell drastically increased the maximum power density and maximum current density to 0.35 mW cm −2 and 4.1 mA cm −2 , respectively, at room temperature (23 °C; Supplementary Fig. S5c ). Elevating the temperature to 50 °C doubled the maximum power density to 0.8 mW cm −2 ( Supplementary Fig. S5d ). The EFC that comprises 13 non-immobilized enzymes based on 15% (wt/v) maltodextrin generated the maximum power density of 0.4 mW cm −2 at a scanning rate of 1 mV s −1 at room temperature. The EFC generated a nearly constant power output of ~0.32 mW cm −2 for 60 h in a closed system ( Fig. 3 ). In addition, a stack of two cuvette-based EFCs can power a digital clock and a light-emitting diode (LED) ( Supplementary Fig. S6 ), suggesting that these EFCs could be used to power a number of electronic devices in the near future. 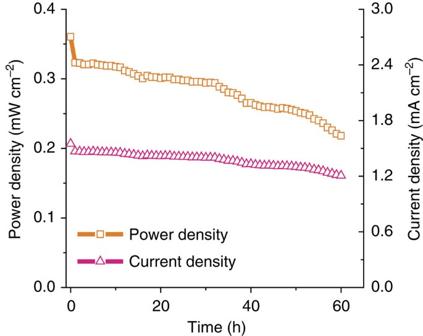Figure 3: Continuous power and current outputs for the 13-enzyme fuel cell. The EFC has an external load of 150 Ω and is run at room temperature. The experimental conditions are 100 mM HEPES, pH 7.5, buffer containing 15% wt/v maltodextrin, 10 mM MgCl2, 0.5 mM MnCl2, 4 mM NAD+, 0.5 mM thiamine pyrophosphate, 40 mM sodium phosphate, 5 mM DTT and non-immobilized enzyme loading conditions of 30 units of 1–4 enzymes, 10 units of 5–12 enzymes, 80 units of DI, 50 mg l−1kanamycin, 40 mg l−1tetracycline, 40 mg l−1cycloheximide, 0.5 g l−1sodium azide, 1 g l−1BSA and 0.1% Triton X-100 in a 15-ml closed anode compartment. Figure 3: Continuous power and current outputs for the 13-enzyme fuel cell. The EFC has an external load of 150 Ω and is run at room temperature. The experimental conditions are 100 mM HEPES, pH 7.5, buffer containing 15% wt/v maltodextrin, 10 mM MgCl 2 , 0.5 mM MnCl 2 , 4 mM NAD + , 0.5 mM thiamine pyrophosphate, 40 mM sodium phosphate, 5 mM DTT and non-immobilized enzyme loading conditions of 30 units of 1–4 enzymes, 10 units of 5–12 enzymes, 80 units of DI, 50 mg l −1 kanamycin, 40 mg l −1 tetracycline, 40 mg l −1 cycloheximide, 0.5 g l −1 sodium azide, 1 g l −1 BSA and 0.1% Triton X-100 in a 15-ml closed anode compartment. Full size image The complete oxidation of the glucose units of the 15% maltodextrin solution means that the energy-storage density of this sugar-powered EFC can be as high as 596 Ah kg −1 , which is more than one order of magnitude higher than the energy-storage densities for lithium-ion batteries and primary batteries ( Fig. 4 and Supplementary Table S3 ). Although the voltages of the EFCs (for example, 0.5 V) are much lower than the voltages of lithium-ion batteries (3.6 V), the energy density of the 15% sugar-powered EFC can reach up to 298 Wh kg −1 , several times that of common rechargeable batteries (for example, Pd acid, NiMH and lithium-ion batteries) and higher than that of common primary batteries (for example, zinc-carbon, alkaline and Li-MnO 2 batteries; Fig. 4 ). The cuvette-based EFC ( Supplementary Fig. S6 ) has an energy-storage density of ~238 Wh kg −1 for the entire system, because the weight of the combined electrode materials, the plastic cuvette and the membrane electrode assembly accounts for ~20% of the entire device weight. Such biobatteries may be regarded as environmentally friendly, disposable primary batteries, because they have better energy densities and less environmental impact. 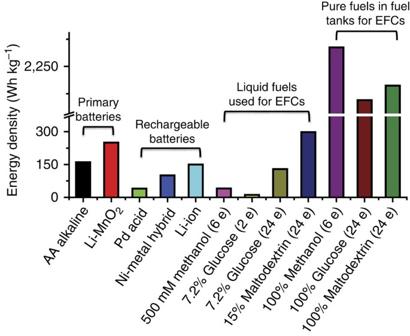Figure 4: Comparison of energy densities among batteries and EFCs. EFCs are powered by 500 mM methanol, 7.2% wt/v glucose or 15% wt/v maltodextrin or dehydrated fuels at a voltage of 0.5 V. More information is available inSupplementary Table S3. Figure 4: Comparison of energy densities among batteries and EFCs. EFCs are powered by 500 mM methanol, 7.2% wt/v glucose or 15% wt/v maltodextrin or dehydrated fuels at a voltage of 0.5 V. More information is available in Supplementary Table S3 . Full size image In addition to the one order-of-magnitude improvement in the energy density of the sugar biobatteries via this synthetic pathway, relative to the system with one redox enzyme ( Fig. 4 ), the biobatteries equipped with non-immobilized enzyme cascades might be refilled by the addition of the sugar solution, because the sole gaseous product (CO 2 ) can be easily released from the anode compartment and the non-immobilized enzymes are not washed out of the EFCs. The non-immobilized enzyme EFC was tested by adding the sugar solution twice ( Supplementary Fig. S7 ). However, the decreased performance of the EFCs suggested more research and development needed for extending the lifetime of EFCs. These sugar biobatteries represent a new type of rechargeable battery. One of the greatest advantages of fuel cells compared with closed primary and secondary batteries is that they are open systems that use high-energy-density fuels (for example, H 2 , methanol, glucose and maltodextrin) that can be fed into the fuel cell device continuously (for example, proton exchange membrane fuel cells) or sporadically (for example, direct methanol fuel cells and sugar batteries [4] , [27] ). When the weight ratio of the fuel to the fuel cell system is large enough (that is, 5–10) or if the fuel cell is refilled a number of times, the energy density of the entire system, including the fuel, a fuel tank and a fuel cell system, can be close to the theoretical energy density of the fuel that is used. Clearly, the use of water-free chemicals as fuels is more attractive in terms of energy-storage density ( Fig. 4 ). However, a separate fuel tank and a complicated fuel feeding system is required in such a system. Maltodextrin is a better EFC fuel than alcohols (for example, methanol) or glucose. Maltodextrin is slowly utilized via the synthetic pathway to generate a nearly constant power output ( Fig. 3 ) rather than a peak power over a short time [10] . In addition, most enzymes cannot work well in high concentrations of alcohol or glucose due to inhibition or low water activity. For example, the highest methanol concentration that can be used in EFCs is ~0.5 M, resulting in a lower energy-storage density of 40.2 Wh kg −1 ( Fig. 4 ) [28] . Similarly, high concentrations of glucose (for example, 0.4 M) [7] lead to high osmotic pressures (~9.85 atm) that can impair enzyme activity [29] . Compared with the six-enzyme EFC that oxidizes glucose to CO 2 (ref. 13 ), the inherently low, but promiscuous, activities of one enzyme that catalyses several substrates results in very low power densities. The use of more than ten enzymes for implementing complex reactions for the production of biocommodities, fine chemicals and pharmaceuticals seems to be not economically prohibitive [25] , [26] , [30] , [31] , [32] , [33] . One of the most important issues for sugar biobatteries is extending their lifetime. This involves improving the stability of enzymes, cofactors and mediators [3] . A preliminary diagnostic experiment was conducted to study the decreased performance of the non-immobilized EFCs ( Supplementary Fig. S8a ). The addition of the new substrate and enzyme mixture to the EFC resulted in a quarter of the maximum power output, suggesting that enzyme deactivation is one of the causes of the decreased power output after more than 1 week of operation at room temperature. Instead of using immobilized enzymes similar to that in most EFCs, we prolonged the lifetime of enzymes using non-immobilized thermoenzymes isolated from (hyper)thermophilic microorganisms [34] . Clearly, relatively non-stable thermoenzymes, such as phosphoglucose isomerase, α-GP and PGM, isolated from thermophiles can be replaced with enzymes from hyperthermophiles or engineered mutant enzymes generated by protein engineering (that is, rational design, directed evolution or a combination of methods). In addition, the half-life time of the non-immobilized enzymes increased from 5.0 days to 7.7 days through the addition of 1 g l −1 BSA and 0.1% Triton X-100 ( Supplementary Fig. S8b ), suggesting that the formulation of enzyme mixture can also be adjusted to prolong the lifetime of non-immobilized enzyme mixtures. Furthermore, replacement of old anodes with new anodes doubles the power output to nearly half of the maximum power output ( Supplementary Fig. S8a ), indicating that leaching of adsorbed VK 3 from the anode results in lower power outputs. Therefore, it will be important to adopt a better method to immobilize VK 3 -like mediators on the surface of anodes [35] . In addition to the enhanced stability of the enzymes and mediators, future research and development on high-power, sugar-powered EFCs should focus on increasing the power density, prolonging the lifetime of the EFCs and replacing the platinum in the cathodes with laccase [8] or bilirubin oxidase [7] . With respect to the first goal, the power density of the EFCs could be increased to 10 mW cm −2 or higher, using a combination of newly developed high-electrical conductivity and high-surface-area nanomaterials as electrodes, such as graphene foams [36] or carbonized nanofibre aerogels [37] , [38] . The performance can also be improved using better mediators [5] , more active enzymes or enzymatic complexes [39] , and optimized enzyme ratios predicted by in silicon models [40] . With respect to the second goal, the use of more stable thermoenzymes, better mediators and cofactors, and better formulation of enzymes can prolong the lifetime of EFCs to months or longer at room temperature, similar to the proteases used in liquid detergents. Moreover, costly and labile NAD can be replaced with low-cost and stable biomimics [41] , [42] . To summarize, high-energy-density sugar biobatteries that use this synthetic catabolic pathway could represent the next generation of environmentally friendly power sources, because of their many appealing features, such as high energy density, safety, biodegradability and low catalyst costs without the need for costly metals and rare earth elements. However, the degradation of EFCs due to the relatively short lifetimes of the enzymes, cofactors and mediators must be resolved before EFCs can be used on a large scale. Chemicals All chemicals, including maltodextrin (dextrose equivalent of 4.0–7.0, that is, a measured degree of polymerization of 19), VK 3 , nicotinamide adenine dinucleotide (NAD, including both the oxidized form (NAD + ) and the reduced form (NADH)), poly- L -lysine (PLL, molecular weight, ~70–150 kDa), dithiothreitol (DTT), 1-(3-dimethylaminopropyl)-3-ethylcarbodiimide hydrochloride (EDC) and N-hydroxysuccinimide were reagent grade or higher and purchased from Sigma-Aldrich (St Louis, MO, USA) or Fisher Scientific (Pittsburgh, PA, USA), unless otherwise noted. Restriction enzymes, T4 ligase and Phusion DNA polymerase were purchased from New England Biolabs (Ipswich, MA, USA). Oligonucleotides were synthesized either by Integrated DNA Technologies (Coraville, IA, USA) or Fisher Scientific. The carbon paper (AvCarb MGL200) used in the anodes was purchased from Fuel Cell Earth (Stoneham, MA, USA). Membrane electrode assemblies consisting of Nafion 212 membranes and a carbon cloth cathode modified with 0.5 mg cm −2 Pt were purchased from Fuel Cell Store (San Diego, CA, USA). COOH-functionalized multiwall CNTs with an outer diameter of <8 nm and a length of 10–30 μm were purchased from CheapTubes.com (Brattleboro, VA, USA). Regenerated amorphous cellulose used in enzyme purification was prepared from Avicel PH105 (FMC, Philadelphia, PA, USA) through its dissolution and regeneration, as described elsewhere [43] . Escherichia coli Top10 was used as a host cell for DNA manipulation and E. coli BL21 Star (DE3) (Invitrogen, Carlsbad, CA, USA) was used as a host cell for recombinant protein expression. Luria–Bertani medium including either 100 mg l −1 ampicillin or 50 mg l −1 kanamycin was used for E. coli cell growth and recombinant protein expression [25] . Production and purification of recombinant enzymes The E. coli BL21 Star (DE3) strain harbouring a protein expression plasmid was incubated in a 1-litre Erlenmeyer flask with 250 ml of the Luria–Bertani medium containing either 100 mg l −1 ampicillin or 50 mg l −1 kanamycin. Cells were grown at 37 °C with rotary shaking at 250 r.p.m. until the absorbance of the cell culture at 600 nm reached 0.6–0.8. Protein expression was induced by adding 100 μM of isopropyl-β- D -thiogalactopyranoside during an 18 °C overnight incubation. The cells were harvested by centrifugation at 4 °C and washed once with 20 mM HEPES (pH 7.5) containing 0.3 M NaCl. The cell pellets were re-suspended in the same buffer and lysed by ultrasonication (Fisher Scientific Sonic Dismembrator Model 500; 5-s pulse on and off, total 300 s at 50% amplitude). After centrifugation, the target proteins in the supernatants were purified. Three approaches were used to purify the various recombinant proteins ( Supplementary Table S1 ). His-tagged proteins were purified by the Profinity IMAC Ni-Charged Resin (Bio-Rad, Hercules, CA, USA). Fusion proteins containing a cellulose-binding-module and self-cleavage intein were purified through high-affinity adsorption on a large-surface-area regenerated amorphous cellulose [44] , [45] . Heat precipitation at 80 °C for 20 min was used to purify ribose-5-phosphate isomerase, ribulose-5-phosphate epimerase, triosephosphate isomerase (TIM) and aldolase [46] , [47] . The purity of the recombinant proteins was examined by SDS–PAGE ( Supplementary Fig. S1 ). Enzyme activity assays Clostridium thermocellum αGP activity was assayed in 100 mM HEPES buffer (pH 7.5) containing 1 mM MgCl 2 , 5 mM DTT, 30 mM maltodextrin and 10 mM sodium phosphate at 23 °C for 5 min. The reaction was stopped with the addition of HClO 4 and neutralized with KOH. Glucose-1-phosphate was measured using a glucose hexokinase/G6PDH assay kit (Pointe Scientific, Canton, MI, USA) supplemented with PGM [6] . C. thermocellum PGM activity was measured in 100 mM HEPES buffer (pH 7.5) containing 5 mM MgCl 2 , 0.5 mM MnCl 2 and 5 mM glucose-1-phosphate at 23 °C for 5 min. The g6p product was determined using a hexokinase/G6PDH assay kit [48] . Geobacillus stearothermophilus G6PDH activity was assayed in 100 mM HEPES buffer (pH 7.5) containing 100 mM NaCl, 2 mM g6p, 2 mM NAD + , 5 mM MgCl 2 and 0.5 mM MnCl 2 at 23 °C. An increase in the absorbance due to the formation of NADH was measured at 340 nm [23] . Morella thermoacetica 6PGDH activity was measured in a 100 mM HEPES buffer (pH 7.5) containing 2 mM 6-phosphogluconate, 2 mM NAD + , 5 mM MgCl 2 and 0.5 mM MnCl 2 at 23 °C for 5 min [23] . Thermotoga maritima ribose-5-phosphate isomerase activity was assayed using a modified Dische’s cysteine–carbazole method [46] . T. maritima ribulose-5-phosphate epimerase activity was determined on a substrate of D -ribulose-5-phosphate as described previously [31] . Thermus thermophilus transketolase activity was measured in a 50 mM Tris/HCl (pH 7.5) buffer containing 0.8 mM D -xylulose 5-phosphate, 0.8 mM D -ribose-5-phosphate, 5 mM MgCl 2 , 0.5 mM thiamine pyrophosphate, 0.15 mM NADH, 60 U ml −1 of TIM and 20 U ml −1 of glycerol 3-phosphate dehydrogenase. The reaction was started with the addition of transketolase at 23 °C. The D -glyceraldehyde 3-phosphate product was quantified through the consumption of NADH measured at 340 nm for 5 min. T. maritima transaldolase activity was assayed as reported previously [49] . T. thermophilus TIM activity was determined in 50 mM Tris/HCl (pH 7.5) containing 5 mM MgCl 2 , 0.5 mM MnCl 2 , 0.5 mg ml −1 BSA, 20 U ml −1 of glycerol 3-phosphate dehydrogenase and 0.25 mM NADH [31] . T. thermophilus fructose-1,6-bisphosphate aldolase was assayed in a 50 mM Tris/HCl buffer (pH 7.5) at 23 °C with 1.9 mM fructose-1,6-bisphosphate as a substrate. The glyceraldehyde 3-phosphate product was quantified with 0.15 mM NADH, 60 U ml −1 of TIM and 20 U ml −1 of glycerol 3-phosphate dehydrogenase at 340 nm [39] . T. maritima fructose-1,6-bisphosphatase activity was determined based on the release of phosphate [45] . C. thermocellum phosphoglucose isomerase activity was assayed at 23 °C in 100 mM HEPES (pH 7.5) containing 10 mM MgCl 2 , 0.5 mM MnCl 2 and 5 mM fructose 6-phosphate [50] . After 3 min, the reaction was stopped with the addition of HClO 4 and neutralized with KOH. The g6p product was analysed at 37 °C with a hexokinase/G6PDH assay kit. G. stearothermophilus DI activity was assayed in 10 mM PBS solution containing 0.16 mM NADH and 0.1 mM dichlorophenolindophenol at 23 °C. A decrease in the absorbance at 600 nm due to the consumption of dichlorophenolindophenol was measured using a spectrometer [23] , [51] . Activities of the G6PDH and DI immobilized on the carbon paper electrodes were assayed under the same conditions as for the free enzymes. The reactions were started by immersing the electrodes in the substrate solution at 23 °C. After removing the electrodes from the reactions, the changes in the absorbance in the reaction solutions were measured as described for the G6PDH and DI assays. Enzyme anode preparation The air-breathing EFC apparatus is shown in Supplementary Fig. S2. The reaction volume of the anode compartment was 15 ml. The electrolyte was deoxygenated by flushing with ultrapure nitrogen for 30 min. The electrolyte was mixed using a magnetic stir bar at 600 r.p.m. The Nafion 212 membrane was used to separate the anode and the cathode whose surface was coated with 0.5 mg cm −2 Pt. The anode compartment was a glass electrolyte container equipped with a rubber stopper for sealing the anode compartment. Two enzyme immobilization methods were used to prepare the anodes equipped with the immobilized enzymes. Method 1 was based on the entrapment of enzymes into a quaternary ammonium-bromide-salt-modified Nafion. The casting solution mixture was prepared by adding 39 mg of TBAB with 1 ml of 5% Nafion 1100 EW suspension (Ion Power, Inc., New Castle, DE, USA). After drying overnight, the mixture was washed with 3.5 ml of 18 MΩ deionized water and re-suspended in 1 ml of isopropanol. The enzyme solution mixture consisted of 1 unit of G6PDH, 40 units of DI, 1 mM NAD + and 0.29 M VK 3 . The carbon paper anode was covered by a mixture of 100 μl of the casting solution and 100 μl of the enzyme solution, and dried at room temperature. Method 2 was based on covalent bond linkage between the enzymes and the CNTs. A 10-μl volume of a 2% wt/v PLL solution was used to coat the carbon paper, followed by addition of 20 μl of 25 mM EDC. Meanwhile, 2.5% wt/v COOH-functionalized CNTs were suspended in a 50% ethanol solution and sonicated for 30 min. The carbon paper was then treated with 40 μl of the CNT-containing solution and dried at room temperature. Another 10 μl of 400 mM EDC and 10 μl of 100 mM N -hydroxysuccinimide were then added, followed by the addition of 1 unit of G6PDH, 40 units of DI, 1 mM NAD + and 10 μl of 0.29 M VK 3 acetone solution. Both types of anodes with immobilized enzymes were stored in 100 mM HEPES buffer containing 2 mM NAD + and 100 mM NaNO 3 at 4 °C before use. For preparation of the non-immobilized enzyme anodes, 1 or 3 mg of CNTs were added to the surface of a 1 cm 2 carbon paper (AvCarb MGL200) from Fuel Cell Earth using PLL (molecular weight, ~70–150 kDa) as described previously [23] . A 10- or 30-μl solution of 0.29 M VK 3 dissolved in acetone was deposited on the dry CNT-containing anode under a hood. After 2 h of acetone evaporation, the water-insoluble VK 3 was deposited onto the anode through physical adsorption. Electrochemical characterization of EFCs All electrochemical tests were performed using a 1000B Multi-Potentiostat (CH Instruments Inc., Austin, TX, USA) interfaced to a personal computer (PC). Experimental data pertaining to current and power outputs were normalized to 1 cm 2 of anode area because the reaction occurring at the anode was the rate-limiting step and the oxidation of protons mediated by Pt in membrane electrode assemblies was not rate limiting. The measurements of open circuit potential and linear sweep voltammetry were performed at a scan rate of 1 mV s −1 . For the comparison of the power generation from the immobilized and non-immobilized enzyme EFCs ( Fig. 1 ), the electrolytes contained 10 mM g6p, 100 mM HEPES buffer (pH 7.5), 2 mM NAD + , 10 mM MgCl 2 and 0.5 mM MnCl 2 . One unit of G6PDH and 40 units of DI were either immobilized on the electrodes or dissolved in the electrolyte. When maltodextrin was used as a substrate ( Fig. 2 ), the electrolytes contained 100 mM HEPES buffer (pH 7.5), non-immobilized enzymes, 0.1 mM maltodextrin, 4 mM NAD + , 4 mM sodium phosphate, 10 mM MgCl 2 , 0.5 mM MnCl 2 , 5 mM DTT and 0.5 mM thiamine pyrophosphate. The one-dehydrogenase EFC contained the first three enzymes plus DI. The two-dehydrogenase EFC contained the first four enzymes plus DI. The EFC used for the complete oxidation of maltodextrin contained all 13 enzymes. The enzyme loading conditions are shown in Supplementary Table S1 . The complete oxidation of maltodextrin was measured ( Fig. 2c and Supplementary Fig. S4 ) in a 100 mM HEPES buffer (pH 7.5) containing 10 mM MgCl 2 , 0.5 mM MnCl 2 , 4 mM NAD + , 4 mM sodium phosphate, 5 mM DTT and 0.5 mM thiamine pyrophosphate. To prevent microbial contamination, 50 mg l −1 kanamycin, 40 mg l −1 tetracycline, 40 mg l −1 cycloheximide and 0.5 g l −1 sodium azide were added. To improve the stability of the enzyme mixture, 1 g l −1 BSA and 0.1% Triton X-100 were added [48] . The enzyme loading conditions are shown in Supplementary Table S1 . Amperometry was conducted at 0 V to achieve the maximal current density. The EFC with 0.2 mM g6p was run for 2 days until nearly zero current was obtained, before a solution of 0.1 mM maltodextrin (that is, ~1.9 mM glucose) was added. The complete oxidation of maltodextrin took ~1 week at room temperature and the remaining maltodextrin was quantified using a SA-20 starch assay kit (Sigma-Aldrich). The Faraday efficiency was calculated according to where F MD−current is the Faraday efficiency, C total is the total charge generated ( C ), Δc glucose unit = c initial −c remain (M), V is reaction volume (l), 24 represents the 24 electrons generated per glucose unit consumed and F is the Faraday constant. The control experiment without maltodextrin was also performed ( Supplementary Fig. S4 ). To further increase the power density of the EFCs, we optimized several factors ( Supplementary Fig. S5 ). The electrolyte was 100 mM HEPES (pH 7.5) buffer containing 20 mM g6p, 10 mM MgCl 2 , 0.5 mM MnCl 2 , 8 mM NAD + , 4 mM sodium phosphate, 0.5 mM thiamine pyrophosphate and G6PDH. All experiments were conducted in the following order: CNT loading (1, 3 or 5 mg per electrode), number of electrode sheets piled up together (1, 3 or 6), enzyme loading (1, 5, 10 or 30 units) and reaction temperature (23, 50, 65 and 80 °C). The best EFC condition was 100 mM HEPES buffer (pH 7.5), 10 mM MgCl 2 , 0.5 mM MnCl 2 , 4 mM NAD + , 0.5 mM thiamine pyrophosphate, 5 mM DTT, 15% (wt/v) maltodextrin, 40 mM sodium phosphate as substrates, and enzyme loading conditions of 30 units of 1–4 enzymes, 10 units of 5–12 enzymes, 80 units of DI, 50 mg l −1 kanamycin, 40 mg l −1 tetracycline, 40 mg l −1 cycloheximide and 0.5 g l −1 sodium azide. For long-term non-disruptive operation, an external resistance of 150 Ω was applied. The power density was measured for 60 h at 23 °C ( Fig. 3 ). How to cite this article: Zhu, Z. A high-energy-density sugar biobattery based on a synthetic enzymatic pathway. Nat. Commun. 5:3026 doi: 10.1038/ncomms4026 (2014).